Quantum computing on encrypted data The ability to perform computations on encrypted data is a powerful tool for protecting privacy. Recently, protocols to achieve this on classical computing systems have been found. Here, we present an efficient solution to the quantum analogue of this problem that enables arbitrary quantum computations to be carried out on encrypted quantum data. We prove that an untrusted server can implement a universal set of quantum gates on encrypted quantum bits (qubits) without learning any information about the inputs, while the client, knowing the decryption key, can easily decrypt the results of the computation. We experimentally demonstrate, using single photons and linear optics, the encryption and decryption scheme on a set of gates sufficient for arbitrary quantum computations. As our protocol requires few extra resources compared with other schemes it can be easily incorporated into the design of future quantum servers. These results will play a key role in enabling the development of secure distributed quantum systems. While quantum computers promise to solve certain classes of problems that are intractable for classical computers [1] , [2] , [3] , [4] , their development is still in its infancy. It is probable that the first quantum computers will act as servers that potential clients can access remotely. In such a server model, the ability to efficiently implement quantum algorithms on encrypted quantum information is crucial. In 2009, the first classical method for fully homomorphic encryption (that is, for performing arbitrary computations over encrypted data) was developed [5] . This enables a client with comparatively little computational power to use an untrusted classical server for performing a computation, without compromising the security of their data. Here we have developed the first scheme for carrying out arbitrary computations on encrypted quantum bits (qubits) where the client only needs to be able to prepare and send single qubits chosen among a set of four possibilities, and to perform some limited classical communication and computation. An important feature of our protocol is that during the computation no quantum communication between the client and the server is required. Strictly speaking, fully homomorphic encryption requires that the client’s total number of operations be proportional to the size of the input and output only. Our scheme satisfies this requirement at the quantum level, but not at the classical one, since the client’s total number of classical operations is proportional to the size of the circuit. Nevertheless, our scheme is efficient, requiring only a constant overhead for performing gates on encrypted data, whereas the best-known fully homomorphic classical solution [6] requires a polylogarithmic overhead. Client–server protocol Our protocol (see Fig. 1 ) starts with a client who has quantum information that needs to be sent to a remote server for processing. The client first encrypts the input qubits. In the circuit model of quantum computing, a universal gate set is required, for example, unitary operations from the Clifford group and one additional non-Clifford gate. For each non-Clifford gate to be performed in the circuit, the client must also prepare an auxiliary qubit according to a prescription we will specify. The client sends the encrypted quantum information and the auxiliary qubits to the server, and the server then sequentially performs the gates specified by the quantum circuit. A round of classical communication between the server and client is required every time a non-Clifford gate is implemented (as shown in Fig. 1h ), allowing the client to update the decryption key. After the algorithm is completed, the server returns the encrypted qubits to the client who then decrypts them. Once decrypted, the client has the answer to the computation the server performed while the server has no knowledge about the quantum information it has processed. The server, however, can choose to perform a different computation. However, for many algorithms of interest [4] , efficient classical verification methods exist, thus enabling the detection of an incorrect output. 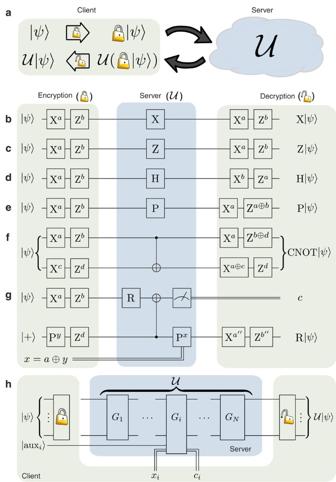Figure 1: Protocol for quantum computing on encrypted data. (a) A client encrypts a quantum stateand sends it to a quantum server, who performs a computationon the encrypted qubit. The server returns the state which the client decrypts to get. (b–g) Encryption and decryption protocols for a universal gate set. Two random classical bitsa,b∈{0,1} (as well asc,d∈{0,1} for the CNOT, (f)) control Pauli rotations X and Z to encrypt state. (b-f) Clifford gates do not require any additional resources and decryption is straightforward. (g) The non-Clifford R gate requires the client to send an auxiliary qubit PyZd, wherey,d∈{0,1}, to control a CNOT gate with the encrypted qubit. The server measures the encrypted qubit and outcomec∈{0,1} is returned to the client, which is used in decryption. The client sends a single classical bit,x=a⊕y, to control a P gate on the auxiliary qubit, which is returned to the client as Xa′′Zb′′R, wherea′′=a⊕candb′′=a(c⊕y⊕1)⊕b⊕d⊕y. (h) For a computation, the client encrypts and sendsto be processed, as well as auxiliary qubits,, for any R gates in the computation. The server performs a series of gates=GN…G1. Communication is only needed when gateGiis an R, and then only with classical bits. Processed qubits are returned to the client for decryption. Figure 1: Protocol for quantum computing on encrypted data. ( a ) A client encrypts a quantum state and sends it to a quantum server, who performs a computation on the encrypted qubit. The server returns the state which the client decrypts to get . ( b – g ) Encryption and decryption protocols for a universal gate set. Two random classical bits a , b ∈ {0,1} (as well as c , d ∈ {0,1} for the CNOT, ( f )) control Pauli rotations X and Z to encrypt state . ( b - f ) Clifford gates do not require any additional resources and decryption is straightforward. ( g ) The non-Clifford R gate requires the client to send an auxiliary qubit P y Z d , where y , d ∈ {0,1}, to control a CNOT gate with the encrypted qubit. The server measures the encrypted qubit and outcome c ∈ {0,1} is returned to the client, which is used in decryption. The client sends a single classical bit, x = a ⊕ y , to control a P gate on the auxiliary qubit, which is returned to the client as X a ′′ Z b ′′ R , where a ′′= a ⊕ c and b ′′= a ( c ⊕ y ⊕ 1) ⊕ b ⊕ d ⊕ y . ( h ) For a computation, the client encrypts and sends to be processed, as well as auxiliary qubits, , for any R gates in the computation. The server performs a series of gates = G N … G 1 . Communication is only needed when gate G i is an R, and then only with classical bits. Processed qubits are returned to the client for decryption. Full size image Our scheme is part of a rapidly developing field that tackles the problem of secure delegated quantum computation. There have been several novel approaches to this problem, including hiding a circuit from the remote quantum server [7] , [8] , computing on encrypted quantum data using multiple rounds and bits of quantum communication [9] , [10] , [11] , [12] and sophisticated methods that provide an additional verification mechanism [10] , [11] , [12] (see Table 1 ). While some of these schemes, in principle, can be used to accomplish similar outcomes as our protocol, they can lead to very different client–server relationships in practice. For example, a recent experiment used the measurement-based model of quantum computing to demonstrate the complementary problem of hiding from a server the circuit that is to be performed [7] , [8] . This method, known as blind quantum computing, can be extended to compute on encrypted data, but would require more than eight times as many auxiliary qubits and significantly more rounds of classical communication. Furthermore, blind computation uses random qubits chosen from a set of eight possibilities—our contribution reduces this to just four. Additionally, our method for computing on encrypted data can be extended to also hide the algorithm from the server via the use of a universal circuit (for details, see Supplementary Note 1 ). Table 1 Comparison with related work. Full size table More fundamentally, blind quantum computing demands a very different relationship between the client and server as compared with our approach that is inspired by homomorphic encryption. In the blind model, the client must provide both the hidden algorithm to be performed and the encrypted data to be computed on; in our scheme the client provides only the data while the server provides the agreed upon algorithm. Our protocol mirrors the client–server relationships that exist today where a server is free to focus on iterating and improving the algorithms they provide. This frees the client from needing to develop and optimize the algorithms they use, while the server is able to specialize in providing targeted services. In the blind model this division of labour does not exist; the server is treated as a ‘dumb’ resource while the client is fully responsible for maintaining and supplying the algorithms. While there are many scenarios where carrying out blind quantum computing is desirable, our protocol enables secure delegated quantum networks to develop in ways that closely resemble today’s networks. In our scheme, to encrypt a qubit , a client applies a combination of Pauli X and Z operations: where a and b are randomly assigned to the values of 0 or 1 and form the key. The action of the encryption maps the initial state of the qubit to one of four possible final states, which sum to the completely mixed state; as long as the values a and b are used only once, this is the quantum equivalent [13] of the classical one-time pad. Knowing a and b , it is possible to decrypt the state by reversing the X and Z rotations. The Clifford gates we study [14] include the single-qubit Pauli X and Z rotations, the two-qubit controlled-NOT (CNOT) gate and the single-qubit Hadamard, , and phase, , gates where j ∈ {0,1}. The actions of the Clifford gates on an encrypted qubit are straightforward due to their commutation relations with the Pauli operators (see Fig. 1b–f ), and do not require any additional classical or quantum resources [9] . The client only needs to know what gates are being carried out to update the knowledge of the decryption key. Clifford gates alone are insufficient for universal quantum computing [15] ; at least one non-Clifford gate is required. We study the non-Clifford R gate, which has the following action: for j ∈ {0,1}. Performing the R gate on encrypted qubits is not trivial as it does not commute through the encryption in the same simple manner as the Clifford gates. This is because the server, when applying the R gate, can introduce an error, equivalent to applying an extra P gate, when a =1: RX a Z b =X a Z a ⊕ b P a R . To prevent the client from needing to divulge the value of a , compromising the security of the computation, the server implements a hidden P gate that is controlled by the client (see Fig. 1g ). To do this, before the server begins the computation the client sends as many auxiliary qubits as there are R gates in the circuit. These auxiliary qubits are encoded as P y Z d with y , d ∈ {0,1}, resulting in one of the four following states that lie along the equator of the Bloch sphere: . These are the four standard BB84 states [16] rotated to a different basis. After the server implements an R gate, it then performs a CNOT between one of the auxiliary qubits and the encrypted state RX a Z b . The server measures the encrypted qubit in the computational basis, and returns the outcome c to the client to update the decryption key. After the CNOT, the state of the auxiliary qubit is X a ′ Z b ′ P a ⊕ y R ; the extra unwanted phase gate now depends on the values of both a and y which only the client knows. The client sends a single classical bit, x = a ⊕ y , which controls whether the server implements an additional corrective P gate without ever revealing the value of a . The final state is then X a ′′ Z b ′′ R as desired, and the decryption key bits, a ′′ and b ′′, now depend on the values of a , b , c , d , and y as shown in the caption for Fig. 1 . A detailed proof of this solution, inspired by circuit manipulation techniques [17] , [18] , is provided in the Supplementary Figs 1–4 and Supplementary Notes 2 and 3 . Also included in Supplementary Note 3 is a novel simulation-based security definition applicable to any untrusted server sharing arbitrary prior information with the client and a proof via an entanglement-based protocol [19] . It is important to note that our security proof assumes the client’s encryption operations are performed perfectly. In Supplementary Note 5 we discuss how imperfections in our experiment affect the security of the protocol. Experimental implementation of the protocol We implement a proof-of-principle of the protocol using linear optics. The state of the qubit is encoded into the polarization of a single photon with horizontal and vertical polarization representing and , respectively. Single photons are generated (see Fig. 2a ) via spontaneous parametric downconversion. The state preparation and encryption, X a Z b , are carried out using a polarizing beamsplitter (PBS), quarter-waveplate (QWP) and half-waveplate (HWP), and the single-qubit Clifford gates are implemented using wave plates (see Fig. 2b ). The CNOT gate (see Fig. 2c ) is implemented using two-photon interference [20] at a partially polarizing beamsplitter (PPBS) [21] , [22] , [23] , which fully transmits horizontally polarized light, but reflects 2/3 of the vertical polarization. 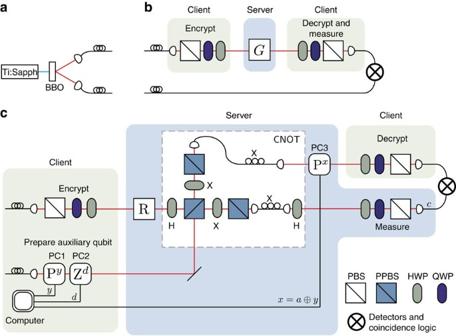Figure 2: Experimental set-up. (a) Photon pairs are generated via spontaneous parametric downconversion using a frequency-doubled Ti:sapphire laser to pump a barium borate (BBO) crystal. Photons are coupled into single-mode fibres. (b) The client prepares and encrypts the qubit, upper rail, using a PBS, QWP and HWP, and then sends it to the server. Single-qubit Clifford gates, shown asG, are implemented as follows: X is a HWP at 45°; Z is a HWP at 0°; H is a HWP at 22.5°; P is a QWP at 0°. The photon is returned to the client, where it is measured using a HWP, QWP and PBS, and detected in coincidence with the second photon from the spontaneous parametric downconversion pair (lower rail). (c) The client prepares and encrypts, upper rail, as inb. The client also prepares an auxiliary photon, lower rail, to one ofusing Pockels’ cells (PC1, PC2) triggered by randomly generated classical bitsyandd. The R gate, a tilted HWP at 0°, acts on photon. Both photons pass through the CNOT, where they interfere at a PPBS. The encrypted photon, in the lower rail, is measured by the server after the CNOT, and the outcomecis used by the client in decryption. The auxiliary photon, now in the upper rail, passes through a third Pockels’ cell (PC3), performing Px, wherex=a⊕yis a classical bit sent from the client, and is returned to the client for decryption and measurement. To test the CNOT gate Pockels’ cells are not used, and state preparation and measurement apparatuses are used in both arms. Figure 2: Experimental set-up. ( a ) Photon pairs are generated via spontaneous parametric downconversion using a frequency-doubled Ti:sapphire laser to pump a barium borate (BBO) crystal. Photons are coupled into single-mode fibres. ( b ) The client prepares and encrypts the qubit , upper rail, using a PBS, QWP and HWP, and then sends it to the server. Single-qubit Clifford gates, shown as G , are implemented as follows: X is a HWP at 45°; Z is a HWP at 0°; H is a HWP at 22.5°; P is a QWP at 0°. The photon is returned to the client, where it is measured using a HWP, QWP and PBS, and detected in coincidence with the second photon from the spontaneous parametric downconversion pair (lower rail). ( c ) The client prepares and encrypts , upper rail, as in b . The client also prepares an auxiliary photon, lower rail, to one of using Pockels’ cells (PC1, PC2) triggered by randomly generated classical bits y and d . The R gate, a tilted HWP at 0°, acts on photon . Both photons pass through the CNOT, where they interfere at a PPBS. The encrypted photon , in the lower rail, is measured by the server after the CNOT, and the outcome c is used by the client in decryption. The auxiliary photon, now in the upper rail, passes through a third Pockels’ cell (PC3), performing P x , where x = a ⊕ y is a classical bit sent from the client, and is returned to the client for decryption and measurement. To test the CNOT gate Pockels’ cells are not used, and state preparation and measurement apparatuses are used in both arms. Full size image To implement the R gate on an encrypted qubit we use an auxiliary qubit along with the CNOT as shown in Fig. 2c . The auxiliary qubit is randomly prepared by the client in one of the four rotated BB84 states, , using waveplates and Pockels’ cells as fast optical switches [24] , [25] , [26] (see Methods ), and then sent to the server. The Pockels’ cells are switched at 1 MHz—two orders of magnitude faster than the single-photon detection rate from spontaneous parametric downconversion. This is done to limit the probability of having multiple photons passing through the Pockels’ cells for the same setting of y and d , reducing the amount of information the server can obtain about the state of the auxiliary qubit, and hence the value of a . The server first performs an R gate on the encrypted qubit followed by a CNOT with the auxiliary qubit. The client then sends the server a classical bit, x = a ⊕ y , which controls whether the server implements an additional corrective P gate using a third Pockels’ cell. Finally, the server returns to the client the encrypted auxiliary qubit containing the final state for processing. In order to characterize our gates we use quantum process tomography [14] , [27] , [28] , [29] ; this provides us with complete information, in the form of a process matrix χ , about how each gate acts on and transforms an arbitrary input state. The client first prepares a set of encrypted input states that the server acts on, and then the client performs measurements on the outputs. For our single-qubit gates the client prepares an overcomplete set of inputs that are the eigenstates of the Paulis . Our encryption scheme, X a Z b , maps each of these Pauli eigenstates into one another. After the server processes the gate, the client performs measurements in each Pauli basis. By choosing this set of input states, and keeping track of the values of a and b , the client is able to completely characterize the action of the gate over all possible encryptions. Similarly, for the two-qubit CNOT gate the client prepares and measures all 36 eigenstates of the tensor products of the Paulis . Again, the encryption scheme maps each of the input eigenstates of the Pauli tensor products into one another, allowing all encryption possibilities to be studied. The client, knowing the decryption key, is able to decrypt and post-process the tomography data. The results for the decrypted single-qubit gates are shown in Fig. 3 and the results for the CNOT are shown in Fig. 4 . The fidelities [14] of the X, Z, H, P, R and CNOT gates are 0.984±0.002, 0.985±0.001, 0.983±0.001, 0.985±0.001, 0.863±0.004 and 0.869±0.004 respectively. Loss of fidelity for single-qubit Clifford gates is predominately due to coherent noise, that is, over- or under-rotation of a unitary, meaning that multiple gates can be performed in sequence maintaining high fidelity. Loss of fidelity for the CNOT and R gates originates from emitted double pairs in the photon source and mode mismatch at the main PPBS. From the client’s perspective, the server has performed the correct computations on the encrypted inputs. However, if the decryption keys are not known, then each gate acts as a completely depolarizing channel that leaves input qubits in the maximally mixed state (as shown in Figs 3 and 4 ). The process matrices were then reconstructed from the same data as before, but without decryption. Each case had high fidelity with the completely depolarizing channel: 0.999±0.001 for the single-qubit gates and 0.996±0.001 for the CNOT. Without knowledge of the decryption keys, the server gains no information about the state . 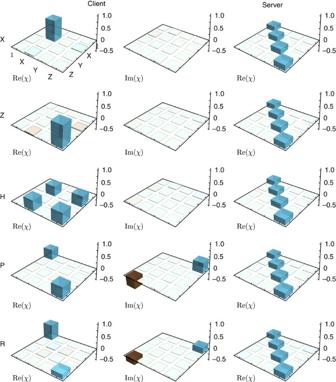Figure 3: Single-qubit gate results. The first two columns, the client, shows real and imaginary parts of reconstructedχmatrices (expressed in the basis of Pauli operators) for the single-qubit gates when decrypted. Fidelities with ideal X, Z, H, P and R gates are 0.984±0.002, 0.985±0.001, 0.983±0.001, 0.985±0.001 and 0.863±0.004, respectively. The third column, the server, shows the real parts (imaginary parts were negligible) of the reconstructedχmatrices when not decrypted, all giving process fidelities of≥0.999 with the completely depolarizing channel. Idealχmatrices are shown inSupplementary Note 4. Figure 3: Single-qubit gate results. The first two columns, the client, shows real and imaginary parts of reconstructed χ matrices (expressed in the basis of Pauli operators) for the single-qubit gates when decrypted. Fidelities with ideal X, Z, H, P and R gates are 0.984±0.002, 0.985±0.001, 0.983±0.001, 0.985±0.001 and 0.863±0.004, respectively. The third column, the server, shows the real parts (imaginary parts were negligible) of the reconstructed χ matrices when not decrypted, all giving process fidelities of ≥0.999 with the completely depolarizing channel. Ideal χ matrices are shown in Supplementary Note 4 . 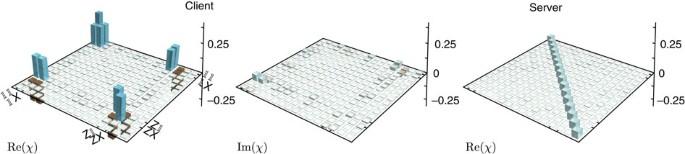Figure 4: CNOT gate results. The first two columns, the client, shows real and imaginary parts of the reconstructed χ matrix for the CNOT gate when the decryption key is known. Fidelity with the ideal CNOT gate is 0.869±0.004. The third column, the server, shows the real part (imaginary part is negligible (<0.004)) of theχmatrix when the key is unknown. The process fidelity with the completely depolarizing channel is 0.996±0.001. Idealχmatrices are shown inSupplementary Note 4. Full size image Figure 4: CNOT gate results. The first two columns, the client, shows real and imaginary parts of the reconstructed χ matrix for the CNOT gate when the decryption key is known. Fidelity with the ideal CNOT gate is 0.869±0.004. The third column, the server, shows the real part (imaginary part is negligible (<0.004)) of the χ matrix when the key is unknown. The process fidelity with the completely depolarizing channel is 0.996±0.001. Ideal χ matrices are shown in Supplementary Note 4 . Full size image Security of the protocol Imperfections in the server’s gates do not affect the security of the protocol, rather just the outcome of the computation. However, imperfections in the client’s encryption and decryption operations do affect the security. We analyse this in Supplementary Note 5 and find that imperfections in the client’s X and Z gates can leak information to the server about the encrypted qubit. Another experimental limitation that impacts the security of the R gate protocol arises from the emission of multiple photon pairs from the source. This can lead to more than one photon being present during a Pockels’ cell setting that is controlled by the bits y and d . The server could potentially use the extra photons to learn the value of the encryption bit a . Based on our source brightness and coupling efficiency we estimate that 22% of the Pockels’ cell settings used contained more than one photon that could be used by the server to break the protocol (see Supplementary Note 5 ). With source development and switching the Pockels’ cells faster, one can improve the security dramatically. For example, if we matched the Pockels’ cells switching rate to the repetition rate of the laser then the number of photons present during each setting can be reduced to 0.6%. One of the key factors in reducing these multi-photon events is to improve the detection efficiency in our system. A primary limitation is the CNOT gate we use, which has a 1/9 success probability. A current theoretical challenge remains to develop more efficient implementations of optical CNOT gates, or alternatively to develop hybrid methods where our photonic qubits can be converted into qubits of another form, that is, ion or microwave qubits, so that the server’s processing can be done on a different architecture more suited to this task. While we make efforts towards quantifying how multi-photon emissions affect the experimental security of the protocol, a complete security analysis is beyond the scope of this current work. In information security often the weakest link is not the transmission of encrypted data, but rather security breaches at the end points where the data is no longer encrypted. A major advance of our scheme is that it eliminates one of the end points as a security risk; a remote server no longer needs to decrypt the quantum information in order to process it and carry out computations. The overhead in quantum resources required to compute on encrypted quantum data is so low (only one auxiliary qubit per non-Clifford gate) that it will be straightforward for future quantum servers to incorporate our protocol in their design, dramatically enhancing the security of client–server quantum computing; our protocol has even less overhead than the best classical fully homomorphic encryption scheme, and provides information-theoretic (as opposed to just computational) security. This method for computing on encrypted quantum data, combined with the techniques developed for quantum circuit hiding [7] , [8] , form a complete security system that will enable secure distributed quantum computing to take place, ensuring the privacy and security of future quantum networks. R gate implementation In the R gate protocol, we initialize auxiliary photons to one of the four states using rubidium titanyl phosphate Pockels’ cells. The values of bits y and d are randomly generated by a computer, and a trigger circuit (based on a self-built CPLD design) is used to drive the Pockels’ cells at a rate of 1 MHz. Single-photon rates are reduced to ~3,800 Hz in the auxiliary qubit path to limit the probability of two photons being present in the Pockels’ cells during a single setting of y and d . Reduced rates also limit the effect of emitted double pairs on the fidelity of the CNOT operation. Photons are detected using silicon avalanche photo-diodes (PerkinElmer four-channel SPCM-AQ4C modules), and coincidence photon events are recorded using a custom design coincidence logic. For all gates, the process that the server observed was attained by summing the measured counts over all the encryption cases a , b ∈ {0,1}. For example, if the client inputs the state , then the server, not knowing the encryption key, would half of the time assume was input and sort the measured counts accordingly. For the R gate the client decrypts by sorting photon counts into eight bins based on the values of y , d and c . The server, not knowing values of y and d , could at most sort counts into two bins based on c , and observes a maximally mixed state due to the active switching, before summing over the encryption key cases. Quantum process tomography Quantum process tomography was performed using a maximum likelihood technique [29] , [30] . Uncertainties in these values are found by adding Poissonian noise to the measured photon counts and performing 100 Monte Carlo iterations of the χ matrix reconstructions. How to cite this article: Fisher, K. A. G. et al . Quantum computing on encrypted data. Nat. Commun. 5:3074 doi: 10.1038/ncomms4074 (2014).